Merotelic attachments allow alignment and stabilization of chromatids in meiosis II oocytes The chromosome segregation process in human oocytes is highly error-prone, generating meiosis II (MII) oocytes with unbalanced chromatids that contribute to aneuploidy in offspring. This raises questions regarding the mechanism for transmission of chromatids and how chromatids evade the error correction mechanisms in MII oocytes. Here, we analyse the behaviour of chromatids in mouse MII oocytes. We find that chromatids align at the spindle equator at the metaphase stage of MII and that their presence does not obstruct entry into the anaphase stage. The alignment process is mediated by merotelic (bi-directional) microtubule–kinetochore attachments, revealing a multi-domain organization of the kinetochore of mammalian meiotic chromosomes. Our results suggest that biorientation of chromatids stabilize microtubule attachments at the kinetochores in a tension-dependent manner. Our results also suggest that merotelic attachments contribute to chromosome mis-segregation in wild-type MII oocytes. Thus, merotely is an important promoter of aneuploidy in mammalian oocytes. An estimated 20% of the oocytes in young women are aneuploid, and this percentage increases with age [1] , [2] . Aneuploidy is a leading genetic cause of miscarriage, congenital birth defects and mental retardation. Most meiotic errors in human oocytes arise due to premature separation of sister chromatids at the first meiotic division, resulting in the formation of meiosis II (MII) oocytes that carry unbalanced (single) chromatids [3] , [4] . To better understand the mechanism through which unbalanced chromatids contribute to aneuploidy, we have taken advantage of a mouse model ( Sycp3 −/− ) in which 30% of the oocytes at the MII stage carry one or a few chromatids [5] . The chromatids in Sycp3 −/− MII oocytes are generated following premature separation of sister chromatids at the first meiotic division and they contribute to the formation of aneuploid embryos [5] , [6] , [7] , [8] . Here we show that chromatids in mouse MII oocytes attain bi-directional microtubule–kinetochore interactions that align them at the spindle equator. This merotelic configuration generates tension that could stabilize microtubules bound to the kinetochore of chromatids, effectively eluding surveillance mechanisms monitoring tension and attachment, and contributing to aneuploidy in mammalian gametes. Chromatids align at the spindle equator in MII oocytes We initially examined the spatial localization of chromatids in cytostatic factor (CSF)-induced metaphase II-arrested mouse oocytes [9] . Wild type and Sycp3 −/− MII oocytes were stained with Hoechst 33342 nuclear dye and analysed using cellular imaging microscopy. We found that the chromosomal material in CSF-induced metaphase II-arrested Sycp3 −/− MII oocytes aligned at the spindle equator ( Fig. 1a ), a surprising result considering that more than 30% of the Sycp3 −/− MII oocytes carry chromatids [5] . Further analysis of fixed CSF-induced metaphase II-arrested Sycp3 −/− MII oocytes stained with 4′,6-diamidino-2-phenylindole (DAPI) and anti-centromeric antiserum (ACA) ACA to respectively label chromatin and centromeres confirmed this result. We found that 90% of the chromatids in Sycp3 −/− MII oocytes localized at the spindle equator ( Fig. 1b,c ), and that 70% of the misaligned chromatids localized close to the spindle equator ( Fig. 1d ). Our results therefore show that chromatids, similar to chromosomes, align at the spindle equator at the metaphase II stage of meiosis in Sycp3 −/− oocytes. 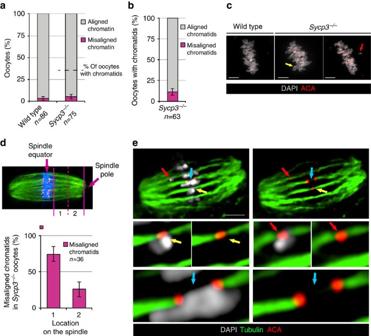Figure 1: Merotelic microtubule–kinetochore attachments promote equatorial alignment of chromatids. (a) Percentage of CSF-arrested meiosis II wild type andSycp3−/−oocytes with chromatin (chromosomes or chromatids) aligned at the spindle equator or misaligned. Chromatin was labelledin vivoby Hoechst 33342 DNA staining. Over 30% of theSycp3−/−MII oocytes contained unbalanced chromatids (indicated by a dashed line5). Data collected from 11 independent experiments. (b) Chromatid localization in fixed MII CSF-arrestedSycp3−/−oocytes. Chromatids were scored as either aligned at the spindle equator or misaligned. Data from 16 independent experiments. (c) Localization of chromosomes and chromatids in fixed MII CSF-arrested wild type andSycp3−/−oocytes. Oocytes were stained with DAPI (DNA staining, grey) and ACA (centromere staining, red). Chromosomes in wild type andSycp3−/−oocytes localized to the spindle equator, whereas chromatids inSycp3−/−oocytes were either aligned at the spindle equator (yellow arrow) or misaligned (red arrow). Images represent a singleZ-plane, corresponding to the focal plane. (d) Localization of misaligned chromatids in fixed MII CSF-arrestedSycp3−/−oocytes. The distance between the outer edge of aligned chromatin at the spindle equator and the spindle pole was divided into two regions (1 and 2) and misaligned chromatids inSycp3−/−oocytes were then categorized into one of the regions. The results are shown as a percentage of all misaligned chromatids. Data from nine independent experiments. (e) Geometry for microtubule–kinetochore attachments for chromosomes and chromatids. Fixed MII CSF-arrestedSycp3−/−oocytes were visualized by using an α-tubulin antibody (green), an anti-centromeric ACA antibody (red) and DAPI to label chromatin (grey), following destabilization of dynamic non-kinetochore microtubules with calcium26. Images shown represent a singleZ-plane. Chromosomes (blue arrow) showed amphithelic attachments with microtubules that protruded into the sister centromeres from opposing sides. Aligned (yellow arrow) and misaligned (red arrow) chromatids displayed microtubules that connected to the single centromeres in a bi-directional (merotelic) manner, representing either end-on or lateral attachments.ndenotes the number of oocytes included in the experiments and vertical bars indicate s.d. (ina,bandd). Bars incanderepresent 10 and 5 μm, respectively. Figure 1: Merotelic microtubule–kinetochore attachments promote equatorial alignment of chromatids. ( a ) Percentage of CSF-arrested meiosis II wild type and Sycp3 −/− oocytes with chromatin (chromosomes or chromatids) aligned at the spindle equator or misaligned. Chromatin was labelled in vivo by Hoechst 33342 DNA staining. Over 30% of the Sycp3 −/− MII oocytes contained unbalanced chromatids (indicated by a dashed line [5] ). Data collected from 11 independent experiments. ( b ) Chromatid localization in fixed MII CSF-arrested Sycp3 −/− oocytes. Chromatids were scored as either aligned at the spindle equator or misaligned. Data from 16 independent experiments. ( c ) Localization of chromosomes and chromatids in fixed MII CSF-arrested wild type and Sycp3 −/− oocytes. Oocytes were stained with DAPI (DNA staining, grey) and ACA (centromere staining, red). Chromosomes in wild type and Sycp3 −/− oocytes localized to the spindle equator, whereas chromatids in Sycp3 −/− oocytes were either aligned at the spindle equator (yellow arrow) or misaligned (red arrow). Images represent a single Z -plane, corresponding to the focal plane. ( d ) Localization of misaligned chromatids in fixed MII CSF-arrested Sycp3 −/− oocytes. The distance between the outer edge of aligned chromatin at the spindle equator and the spindle pole was divided into two regions (1 and 2) and misaligned chromatids in Sycp3 −/− oocytes were then categorized into one of the regions. The results are shown as a percentage of all misaligned chromatids. Data from nine independent experiments. ( e ) Geometry for microtubule–kinetochore attachments for chromosomes and chromatids. Fixed MII CSF-arrested Sycp3 −/− oocytes were visualized by using an α-tubulin antibody (green), an anti-centromeric ACA antibody (red) and DAPI to label chromatin (grey), following destabilization of dynamic non-kinetochore microtubules with calcium [26] . Images shown represent a single Z -plane. Chromosomes (blue arrow) showed amphithelic attachments with microtubules that protruded into the sister centromeres from opposing sides. Aligned (yellow arrow) and misaligned (red arrow) chromatids displayed microtubules that connected to the single centromeres in a bi-directional (merotelic) manner, representing either end-on or lateral attachments. n denotes the number of oocytes included in the experiments and vertical bars indicate s.d. (in a , b and d ). Bars in c and e represent 10 and 5 μm, respectively. Full size image Chromatid alignment is supported by merotelic attachments What promotes equatorial alignment of chromatids at the metaphase II stage in Sycp3 −/− oocytes? To answer this question, we analysed the nature of the microtubule–kinetochore interactions for chromosomes and chromatids in CSF-induced metaphase II-arrested Sycp3 −/− oocytes. We found that chromosomes at the spindle equator displayed an amphitelic configuration ( Fig. 1e ), a geometric orientation promoted by opposing end-on microtubule attachments to the sister kinetochores of chromosomes [10] , [11] , [12] . Occasionally, one of the two sister kinetochores of chromosomes were bi-directionally attached to microtubules, suggesting also the presence of merotelic attachments ( Supplementary Fig. 1 ). Importantly, chromatids localized at the spindle equator displayed bi-directional attachments, in this situation involving a single kinetochore only, generating a merotelic configuration ( Fig. 1e ). Analysis of chromatids localized at an intermediary position in between the pole and the equator of the spindle ( Fig. 1e , Supplementary Fig. 2 ) revealed that these also were in contact with microtubules, either through bi-directional attachments or through lateral surface interactions. Thus, our results strongly suggest that lateral interactions and merotelic attachments contribute to congression and biorientation of chromatids at the metaphase stage of MII in oocytes. Chromatid attachments contribute to spindle assembly checkpoint silencing End-on attachment of microtubules to the kinetochores of chromosomes reduces Mad2 levels at kinetochores and contributes to silencing of the spindle assembly checkpoint (SAC) in mitotic and meiotic cells [13] , [14] , [15] . To find out whether the level of Mad2 was different at the kinetochores of chromosomes and chromatids, Sycp3 −/− oocytes arrested at the metaphase II stage were labelled using an antibody against Mad2. We found the relative intensity of the Mad2 signal at kinetochores to be identical for chromosomes and chromatids ( Fig. 2a,c ). Importantly, treatment of metaphase II-arrested oocytes with nocodazole (a spindle poison that depolymerizes microtubular filaments and abolishes their attachments to the kinetochores) resulted in a strongly increased Mad2 signal at the kinetochores of both chromatids and chromosomes ( Fig. 2a,c ). We also measured the relative intensity of the Mad2 signal at the kinetochores of chromosomes and chromatids in Sycp3 −/− oocytes that were first released from CSF-induced metaphase II arrest by adding strontium. Again, we found that the Mad2 signal had the same intensity on the kinetochores of both chromatids and chromosomes, both in the presence and in the absence of nocodazole ( Fig. 2b,d ). These results suggest that merotelic end-on attachments to the kinetochores of chromatids silence Mad2-signalling and contribute to SAC inactivation at the metaphase II stage in Sycp3 −/− oocytes. 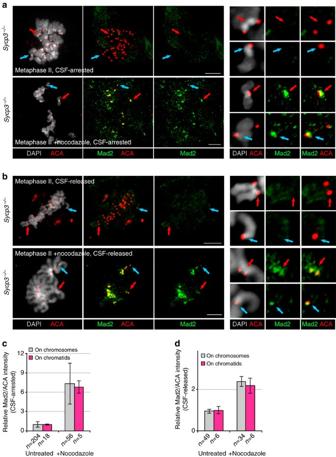Figure 2: Mad2 levels at the kinetochores of chromatids and chromosomes are identical. (a,b) Mad2 localization at kinetochores of chromosomes and chromatids was analysed in fixedSycp3−/−CSF-arrested MII oocytes (a) or inSycp3−/−metaphase II oocytes released from CSF arrest (90 min after addition of strontium) (b). Staining was performed in the presence or absence of nocodazole. Mad2 was labelled using an antibody (green), centromeres labelled by an ACA antibody (red) and chromatin stained by DAPI (grey). Individual representative chromosomes and chromatids (indicated by red and blue arrows, respectively) were separately magnified to visualize the Mad2 (green) and ACA (red) signals. Scale bars, 10 μm. (c,d) Relative Mad2 levels at kinetochores of chromosomes and chromatids were analysed in fixedSycp3−/−CSF-arrested MII oocytes (c) or inSycp3−/−MII oocytes released from CSF arrest (90 min after addition of strontium) (d). Mad2 levels were calculated from the relative intensity of the Mad2/ACA antibody signals at kinetochores of chromosomes (grey) and chromatids (red). Staining was performed in the presence or absence of nocodazole. The relative intensity values were normalized for the chromosomes to a value of 1.ndenotes the number of analysed chromosomes or chromatids, data collected from three independent experiments. Error bars indicate s.d. Figure 2: Mad2 levels at the kinetochores of chromatids and chromosomes are identical. ( a , b ) Mad2 localization at kinetochores of chromosomes and chromatids was analysed in fixed Sycp3 −/− CSF-arrested MII oocytes ( a ) or in Sycp3 −/− metaphase II oocytes released from CSF arrest (90 min after addition of strontium) ( b ). Staining was performed in the presence or absence of nocodazole. Mad2 was labelled using an antibody (green), centromeres labelled by an ACA antibody (red) and chromatin stained by DAPI (grey). Individual representative chromosomes and chromatids (indicated by red and blue arrows, respectively) were separately magnified to visualize the Mad2 (green) and ACA (red) signals. Scale bars, 10 μm. ( c , d ) Relative Mad2 levels at kinetochores of chromosomes and chromatids were analysed in fixed Sycp3 −/− CSF-arrested MII oocytes ( c ) or in Sycp3 −/− MII oocytes released from CSF arrest (90 min after addition of strontium) ( d ). Mad2 levels were calculated from the relative intensity of the Mad2/ACA antibody signals at kinetochores of chromosomes (grey) and chromatids (red). Staining was performed in the presence or absence of nocodazole. The relative intensity values were normalized for the chromosomes to a value of 1. n denotes the number of analysed chromosomes or chromatids, data collected from three independent experiments. Error bars indicate s.d. Full size image Lagging chromosomes at anaphase in wild-type MII oocytes To further investigate the process through which chromatids congress and segregate in MII oocytes, we used live-cell time-lapse microscopy to track individual chromosomes and chromatids throughout cell division in MII oocytes. Wild type and Sycp3 −/− mice were crossed with a mouse strain that carries an integrated H2B-mCherry transgene, generating female mice that expresses a fluorescent histone fusion protein in oocytes. H2B-mCherry-expressing wild type and Sycp3 −/− oocytes were released from CSF-induced metaphase II arrest by strontium and then monitored by live-cell imaging through the second meiotic division. We found that most wild-type MII oocytes underwent an error-free cell division process ( Fig. 3a,b ; Supplementary Videos 1–4 ). Further analysis revealed that approximately 20% of the wild-type MII oocytes displayed transient chromosome misalignments, errors that were corrected before anaphase onset ( Fig. 3a,b ). Importantly, 9% of the wild-type MII oocytes contained lagging chromosomes at anaphase onset, suggesting that merotelic microtubule–kinetochore attachments contribute significantly to chromosome mis-segregation events in wild-type MII oocytes. 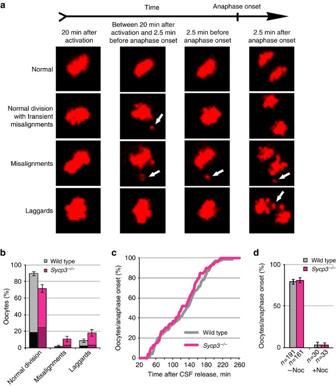Figure 3:Sycp3−/−oocytes with chromatids display an increased level of segregation defects, but their entry into anaphase is not obstructed. (a) Chromosome and chromatid segregation patterns in mouse MII CSF-released oocytes were identified by time-lapse imaging every 2.5 min. The columns from left to right show four different time points following CSF release. In a normal MII division (upper row), the chromosomes localized as a single chromatin structure at the metaphase plate and segregated into two separate chromatin structures. We observed in both wild type andSycp3−/−metaphase II oocytes three types of deviating patterns, including transient misalignments (second row), misalignments that persisted at anaphase onset (third row) and chromatin that remained at the spindle midzone at anaphase onset (laggards, bottom row). Arrows indicate chromatin fragments, corresponding to chromosomes or chromatids. (b) Quantification of chromosome and chromatid segregation patterns in mouse oocytes. Time-lapse imaging was performed for 150 wild type (grey) and 84Sycp3−/−(red) MII oocytes following release from CSF arrest and the segregation pattern for individual cells categorized into one of three categories. Transient misalignments observed in cells categorized into one of the three categories are shown in black (for wild-type oocytes) or in dark red (forSycp3−/−oocytes). Data from seven independent experiments. Error bars indicate s.d. (c) Cumulative curves for the time of anaphase onset in wild type (grey line,n=150) andSycp3−/−(red line,n=84) MII oocytes, released from CSF arrest. The vertical axis shows the cumulative percentage of all oocytes that entered anaphase, while the horizontal axis indicates the time after CSF release, in minutes. Data from seven independent experiments. (d) Efficiency in entering anaphase. Wild type andSycp3−/−MII oocytes were released from CSF arrest in the presence or absence of nocodazole and monitored by live-cell imaging. The percentage of wild type (grey bars) andSycp3−/−(red bars) MII oocytes that entered anaphase was identical. Nocodazole blocked anaphase onset for both wild type (grey bars) andSycp3−/−(red bars) MII oocytes.ndenotes the number of oocytes included in the experiments. Error bars indicate s.d. Data from three independent experiments. Figure 3: Sycp3 −/− oocytes with chromatids display an increased level of segregation defects, but their entry into anaphase is not obstructed. ( a ) Chromosome and chromatid segregation patterns in mouse MII CSF-released oocytes were identified by time-lapse imaging every 2.5 min. The columns from left to right show four different time points following CSF release. In a normal MII division (upper row), the chromosomes localized as a single chromatin structure at the metaphase plate and segregated into two separate chromatin structures. We observed in both wild type and Sycp3 −/− metaphase II oocytes three types of deviating patterns, including transient misalignments (second row), misalignments that persisted at anaphase onset (third row) and chromatin that remained at the spindle midzone at anaphase onset (laggards, bottom row). Arrows indicate chromatin fragments, corresponding to chromosomes or chromatids. ( b ) Quantification of chromosome and chromatid segregation patterns in mouse oocytes. Time-lapse imaging was performed for 150 wild type (grey) and 84 Sycp3 −/− (red) MII oocytes following release from CSF arrest and the segregation pattern for individual cells categorized into one of three categories. Transient misalignments observed in cells categorized into one of the three categories are shown in black (for wild-type oocytes) or in dark red (for Sycp3 −/− oocytes). Data from seven independent experiments. Error bars indicate s.d. ( c ) Cumulative curves for the time of anaphase onset in wild type (grey line, n =150) and Sycp3 −/− (red line, n =84) MII oocytes, released from CSF arrest. The vertical axis shows the cumulative percentage of all oocytes that entered anaphase, while the horizontal axis indicates the time after CSF release, in minutes. Data from seven independent experiments. ( d ) Efficiency in entering anaphase. Wild type and Sycp3 −/− MII oocytes were released from CSF arrest in the presence or absence of nocodazole and monitored by live-cell imaging. The percentage of wild type (grey bars) and Sycp3 −/− (red bars) MII oocytes that entered anaphase was identical. Nocodazole blocked anaphase onset for both wild type (grey bars) and Sycp3 −/− (red bars) MII oocytes. n denotes the number of oocytes included in the experiments. Error bars indicate s.d. Data from three independent experiments. Full size image Segregation errors in MII oocytes with chromatids We next monitored H2B-mCherry-expressing Sycp3 −/− oocytes that first were released from CSF-induced metaphase II arrest by strontium and then monitored by live-cell imaging through the second meiotic division. We found that Sycp3 −/− MII oocytes, relative to wild-type MII oocytes, displayed a slightly increased level of transient misalignments, as well as a twofold increased level of laggards at anaphase onset ( Fig. 3a,b ). To better understand the nature of the transient misalignments, these were further studied in more detail in individual oocytes. We found that transient misalignments at different time points during the second meiotic division were present in a larger fraction of Sycp3 −/− oocytes compared with wild-type oocytes ( Fig. 4a ). The increased presence of transient misalignments in Sycp3 −/− MII oocytes was found to be owing to two cumulative factors: 1, that misalignments required more time for re-alignment at the equator ( Fig. 4b ), and 2, that misalignments occurred more frequently in a consecutive way in individual Sycp3 −/− MII oocytes ( Fig. 4c ). At anaphase onset, 10% of Sycp3 −/− MII oocytes retained misalignments—a segregation defect observed in approximately 2% of the wild-type MII oocytes ( Fig. 3b ). The increased presence of laggards and misalignments identified in Sycp3 −/− MII oocytes (relative to wild-type MII oocytes) most likely relates to the presence of chromatids in mutant oocytes. 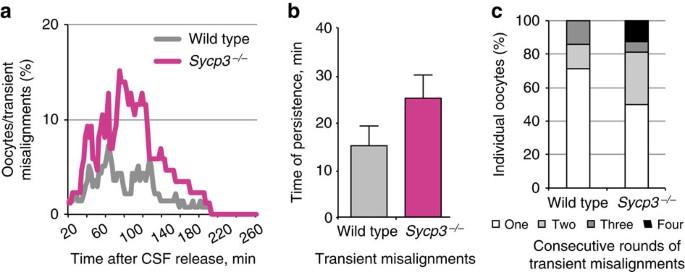Figure 4: Transient misalignments take place at an increased rate and remain uncorrected for longer period of time inSycp3−/−CSF-released MII oocytes. (a) Transient misalignments are frequently observed inSycp3−/−MII oocytes. Occurrence of transient misalignments in wild type (grey line) andSycp3−/−(red line) MII oocytes following the release from CSF arrest, shown as percentage of all oocytes that initiated anaphase. The vertical axis shows the percentage of oocytes that displayed transient misalignments at each time point, while the horizontal axis indicates the time after release from CSF arrest, in minutes. (b) Transient misalignments persist longer inSycp3−/−oocytes. Persistence of transient misalignments was measured in wild type andSycp3−/−MII oocytes following the release from CSF arrest (P=0.03, Mann–Whitney test). The average time of persistence for transient misalignments was 15 min in wild-type oocytes (grey column,n=31), versus 25 min forSycp3−/−oocytes (red column,n=23). Vertical axis shows time in minutes, error bars indicate s.e.m. (c) Transient misalignments appear in a consecutive manner in individualSycp3−/−oocytes. The number of sequential transient misalignments was determined in wild type (n=28) andSycp3−/−(n=17) MII oocytes following the release from CSF arrest. The grey scale within the columns indicates the number of consecutive rounds that transient misalignments appeared in individual oocytes. Data from seven independent experiments. Figure 4: Transient misalignments take place at an increased rate and remain uncorrected for longer period of time in Sycp3 −/− CSF-released MII oocytes. ( a ) Transient misalignments are frequently observed in Sycp3 −/− MII oocytes. Occurrence of transient misalignments in wild type (grey line) and Sycp3 −/− (red line) MII oocytes following the release from CSF arrest, shown as percentage of all oocytes that initiated anaphase. The vertical axis shows the percentage of oocytes that displayed transient misalignments at each time point, while the horizontal axis indicates the time after release from CSF arrest, in minutes. ( b ) Transient misalignments persist longer in Sycp3 −/− oocytes. Persistence of transient misalignments was measured in wild type and Sycp3 −/− MII oocytes following the release from CSF arrest ( P =0.03, Mann–Whitney test). The average time of persistence for transient misalignments was 15 min in wild-type oocytes (grey column, n =31), versus 25 min for Sycp3 −/− oocytes (red column, n =23). Vertical axis shows time in minutes, error bars indicate s.e.m. ( c ) Transient misalignments appear in a consecutive manner in individual Sycp3 −/− oocytes. The number of sequential transient misalignments was determined in wild type ( n =28) and Sycp3 −/− ( n =17) MII oocytes following the release from CSF arrest. The grey scale within the columns indicates the number of consecutive rounds that transient misalignments appeared in individual oocytes. Data from seven independent experiments. Full size image Chromatids do not delay entry into anaphase II We then asked if the segregation defects in Sycp3 −/− MII oocytes obstructed the ability of these cells to complete the second meiotic division. We found, however, that Sycp3 −/− MII oocytes entered into the anaphase stage with a similar temporal profile and as efficiently as wild-type oocytes ( Fig. 3c,d ). This result cannot be explained by the presence of an impaired SAC in Sycp3 −/− MII oocytes, as nocodazole inhibited anaphase onset with similar efficiency in wild type and mutant oocytes ( Fig. 3d ). We conclude that neither the presence of single chromatids nor an increased level of segregation errors affected the ability of Sycp3 −/− MII oocytes to complete the second meiotic division. We show here that a large majority of the chromatids in Sycp3 −/− MII oocytes align at the spindle equator at the metaphase stage, displaying merotelic microtubule–kinetochore attachments. This result is in agreement with previous studies of the behaviour of chromatids in mammalian somatic cells and in plant meiotic cells [16] , [17] , [18] , [19] . These studies showed that mammalian and plant kinetochores are organized into multiple domains, promoting the formation of bi-directional microtubule attachments at the kinetochores of chromatids [17] , [18] . An important question arising from these studies is why merotelic, and not monotelic, attachments are established at the kinetochores of chromatids? In both geometric orientations, the attachments to the kinetochores should contribute to the silencing of the SAC [19] , [20] . We find, however, very rarely chromatids to be localized to the spindle poles in Sycp3 −/− MII oocytes, which would be the predicted localization of chromatids resulting from a monopolar attachment. Syntelic attachments (analogous to the monopolar attachments for chromatids) are effectively replaced by amphitelic attachments (analogous to the merotelic attachments for chromatids) in somatic cells during mitosis [19] , [20] . This is likely a consequence of the fact that amphitelic, but not syntelic attachments, generates intra- and inter-kinetochore tension, tension that increases the number of microtubules bound to kinetochores and stabilize their interactions [21] , [22] , [23] . We propose that the merotelic attachments observed at chromatids in Sycp3 −/− MII oocytes fulfil a role similar to that of amphitelic attachments for chromosomes, generating tension across the single kinetochore of chromatids and contributing to microtubule recruitment and stabilization. Formation of merotelic attachments at chromatids could be of particular importance in acentriolar meiotic cells, where tension at kinetochores cannot be established through polar ejection forces [24] , [25] , [26] . The biorientation process of chromatids in Sycp3 −/− MII oocytes is likely to be promoted by lateral gliding of chromatids towards the spindle equator, as shown for somatic cells [24] , [25] , [26] . The fact that we see very few chromatids close to the poles in Sycp3 −/− MII oocytes strongly suggests that tension, resulting from merotelic attachments, effectively contributes to alignment and stabilization of chromatids at the spindle equator. Tension established though bi-directional attachment of chromatids should help to maintain SAC inactivation and to elude surveillance mechanism monitoring attachment and tension, promoting chromatid transmission and formation of aneuploid gametes. The CSF arrest that precedes activation and anaphase entry in MII oocytes could provide time for establishing merotelic attachments for chromatids, as SAC is not essential for maintaining CSF arrest in mouse oocytes [9] . Importantly, we have found that also wild-type MII oocytes frequently display merotelic attachments at the metaphase stage, as well as lagging chromosomes at anaphase onset. This strongly suggests that merotelic attachments contribute significantly to chromosome mis-segregation in wild-type female germ cells, similar to what previously been documented for somatic cells during mitosis [10] , [11] , [27] . In conclusion, our results show that merotely contributes to aneuploidy in mammalian oocytes. Animal studies The animal experiments were approved by the Stockholm-North Animal Ethical Committee. Oocytes were taken from 3–4-week or 11–13-week old female mice carrying a null mutation for the Sycp3 gene and their wild-type siblings, produced on the mixed C57BL/6NCrl × 129/OlaIHsd background [6] . Ovaries from wild type and Sycp3 −/− mice were dissected and the oocytes at the germinal vesicle stage were released with the 26G needle into M2 medium (Sigma). Oocytes that underwent germinal vesicle breakdown within 2 h were further matured for 13–14 h at 37 °C. Oocytes that extruded the polar body and arrested in a CSF-dependent manner at the metaphase II stage were released from cumulus cells by pipetting and used for further studies. Oocytes were activated through incubation in Ca 2+ -free potassium simplex optimization medium (KSOM) media supplemented with 10 mM SrCl 2 . For visualization of chromatin alignment, live oocytes were stained with 1 μg ml −1 Hoechst 33342 (Invitrogen) and images captured at × 10 magnification on a Leica DMRXA microscope. Immunofluorescence microscopy Cumulus-free CSF-arrested were fixed immediately following their collection, and activated oocytes were fixed 90 min after their release into strontium-containing activation medium. In brief, oocytes were incubated 3 min in Tyrode’s solution (Sigma) to remove zone pellucida and dropped on a slide dipped in 1% paraformaldehyde/0.15% Tritoin X-100. The slides were air-dried for 2 h, rehydrated in phosphate-buffered saline (PBS)/0.01% Triton X-100 and then blocked for 1 h in 3% bovine serum albumin in PBS/0.01% Triton X-100. In total, 400 nM nocodazole (Sigma) was added to the M2 media or to the Ca 2+ -free KSOM medium with SrCl 2 for 60–100 min. Visualization of microtubule–kinetochore geometry was done in intact CSF-arrested oocytes. Microtubules were destabilized in Ca 2+ buffer (100 mM PIPES pH 7.0, 1 mM MgCl 2 , 0.1 mM CaCl 2 , 0.1% Triton X-100) for 90 s and fixed with 1% formaldehyde in the Ca 2+ buffer for 30 min at room temperature. After the fixation, the oocytes were washed with PBS/0.1% Triton X-100 four times, extracted overnight at 4 °C, and then blocked with 3% bovine serum albumin in PBS/0.01% Triton X-100 for 1 h at room temperature. The following antibodies and dilutions were used for immunolocalization studies: human ACA antiserum 1:200 (Antibodies, Cat# 15-234-0001), rabbit anti-MAD2 1:50 (Covance, Cat #PRB-452C) and mouse anti-α-tubulin 1:200 (Sigma, Cat# T-9026). Secondary antibodies used were swine-anti-rabbit FITC (DAKO) 1:400, donkey anti-mouse Alexa488 (Invitrogen) 1:1,000, goat-anti-human Cy5 (Amersham) 1:3,000 and goat-anti-human Cy3 (Amersham) 1:1,000. Spread oocytes after staining were mounted in Prolong Gold mounting medium containing DAPI (Molecular Probes) and a single image representing the focal plane was captured using Leica DMRXA microscope at × 1,000 magnification. The entire spindle in fixed intact oocytes was imaged at × 1,000 magnification every 0.2 μm using a DeltaVision microscope (Applied Precision). Images were processed using Openlab 3.1.4 software (Improvision), Volocity 6.0 software (Perkin Elmers), SoftWoRx 3.3.1 software (DeltaVision) and Adobe Photoshop 8.0. For quantification of signals on the kinetochores, the centromeric regions as defined by ACA signal were outlined and the integrated density of Mad2 and ACA signals on single chromatids and chromosomes were calculated using ImageJ software. The average ratio Mad2/ACA at chromosomes without nocodazole were normalized to 1 and thereafter compared with the values for the chromatids. To minimize the variability in quantification of following nocodazole treatment, oocytes incubated with and without nocodazole were fixed on the same slide. Time-lapse imaging A reporter gene, coding for histone H2B fused to a mCherry fluorescent molecule, was introduced into the experimental mouse strain by backcrossing with reporter mice carrying a H2B-mCherry fusion gene [28] . Time-lapse imaging of oocytes undergoing second meiotic division was performed in Ca 2+ -free KSOM medium supplemented with 10 mM of SrCl 2 using a Leica DMI6000 microscope at 37 °C, 5% CO 2 . Red fluorescence and differential contrast (DIC) images were captured every 2.5 min at × 20 magnification for 4 h, for a total of 20–25 1.5-μm Z-sections. For the nocodazole assay, oocytes were imaged in the M2 or Ca 2+ -free KSOM medium with SrCl 2 supplemented with 400 nM nocodazole (Sigma) for 4 h. Oocytes that degraded during that period were excluded from further analysis. The first time frame when chromatin showed a bi-directional poleward movement was scored as anaphase onset. Misalignments in oocytes were scored when smaller chromatin bodies became visibly separated from the central chromatin mass. Experiments involving Sycp3 −/− oocytes were always performed in parallel with wild-type oocytes. Statistical analysis Statistical analysis was performed using Prism 6 software. How to cite this article: Kouznetsova, A. et al. Merotelic attachments allow alignment and stabilization of chromatids in meiosis II oocytes. Nat. Commun. 5:4409 doi: 10.1038/ncomms5409 (2014).